Cis-andtrans-regulatory divergence between progenitor species determines gene-expression novelty inArabidopsisallopolyploids Gene-expression divergence between species shapes morphological evolution, but the molecular basis is largely unknown. Here we show cis - and trans -regulatory elements and chromatin modifications on gene-expression diversity in genetically tractable Arabidopsis allotetraploids. In Arabidopsis thaliana and Arabidopsis arenosa , both cis and trans with predominant cis -regulatory effects mediate gene-expression divergence. The majority of genes with both cis - and trans -effects are subjected to compensating interactions and stabilizing selection. Interestingly, cis - and trans -regulation is associated with chromatin modifications. In F1 allotetraploids, Arabidopsis arenosa trans factors predominately affect allelic expression divergence. Arabidopsis arenosa trans factors tend to upregulate Arabidopsis thaliana alleles, whereas Arabidopsis thaliana trans factors up- or down-regulate Arabidopsis arenosa alleles. In resynthesized and natural allotetraploids, trans effects drive expression of both homoeologous loci into the same direction. We provide evidence for natural selection and chromatin regulation in shaping gene-expression diversity during plant evolution and speciation. Interspecific hybridization and polyploidy occur in many flowering plants and some animals, leading to novel phenotypic variation [1] , [2] , [3] , [4] , [5] . Barbara McClintock [6] coined the term 'genome shock' to describe unprepared changes to cope with an existing programmed response in interspecific hybrids, leading to transposon activation and genomic instability. Recent studies have shown that genome hybridization between species also induces novel changes in gene-expression 'shock', as observed in many allopolyploids including Arabidopsis [7] , cotton [8] , and Senecio [9] . The induced variation in the interspecific hybrids can be transmitted to the progeny if chromosomes are doubled to form stable allopolyploids [5] , [10] . Genome hybridization and polyploidization have had a pervasive role in the evolution and domestication of many flowering plants including the most important crops such as wheat, cotton and canola [2] , [3] , [4] , [10] . Gene-expression differences between parental alleles or homoeologs can result from cis - and/or trans -regulatory changes. Changes in cis -regulatory elements and transcribed regions affect transcription and messenger RNA stability [11] , [12] . Trans effects could result from functional divergence of transcription factors and chromatin regulators or from other components that transduce environmental signals into gene-expression changes. Cis and trans effects have been documented in intra- and inter-specific hybrids of Drosophila [11] , [13] , yeast [12] , maize [14] , maize aneuploids [15] and an aneuploid mouse strain carrying a human chromosome 21 [16] . The results suggest predominant cis effects on expression divergence between species, whereas trans regulation is often associated with cis -regulation and sensory responses to the environment. However, recent evidence indicates that gene-expression stability is maintained by coordinated cis - and trans -regulatory activities [17] , [18] . Changes in both cis - and trans -regulatory elements are responsible for the maintenance of the overall expression circuits [18] and coevolution between a DNA-binding transcription factor and its cis -binding site [19] . Studies on cis - and trans -regulation are often performed in F1 interspecific hybrids [11] , [12] , [13] or in somatic hybrid (mouse-human) cells that carry one or more alien chromosomes [16] . Many interspecific hybrids cannot produce offspring, so it is difficult to test consequences of cis - and trans -regulation on phenotypes. Somatic hybrid cell lines are immortal, but the information derived from these lines is not directly relevant to physiology and behaviour at the organismal level. To overcome these caveats, we have developed a plant model system for the study. We resynthesized multiple allotetraploid lineages between Arabidopsis thaliana autotetraploid and Arabidopsis arenosa tetraploids [7] , [20] , [21] . These allotetraploid lines are genetically stable and tractable and suitable for this study. Here we employed mRNA (cDNA) sequencing (RNA-seq) analysis to investigate relative contributions of cis - and trans regulation to gene-expression divergence between the two related species, the expression novelty of homoeologous genes in resynthesized allotetraploids, and the inheritance and maintenance of altered expression patterns in stable and natural allotetraploids. Dominant cis effects on gene-expression divergence Arabidopsis allotetraploids were formed between A. thaliana and A. arenosa, the two species that diverged ~6 million years ago [22] ( Fig. 1a ). The resynthesized allotetraploids (F1) were self-pollinated to generate allotetraploid lines (F8) [7] , [20] , [21] , and they are comparable with the natural allotetraploid Arabidopsis suecica [23] . Cis - and trans -effects of gene-expression changes between these related Arabidopsis species were determined using RNA-seq analysis with Illumina G2 and HiSeq 2000 in rosette leaves collected before bolting (Methods). For F1 allotetraploids and their progenitors, each of three biological replicates consisted of 12–19 million sequencing reads. For F8 allotetraploids and natural A. suecica , 12–57 million sequence reads were generated ( Supplementary Fig. S1 and Supplementary Table S1 ). 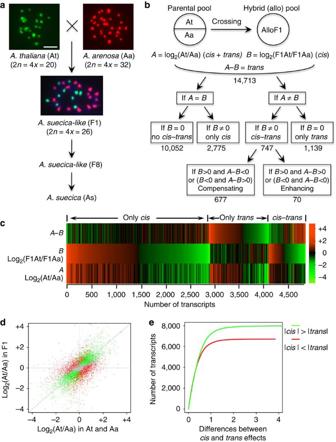Figure 1:Arabidopsisallotetraploids progenitors and distribution of genes withcisandtranseffects. (a) Fluorescencein situhybridization images ofA. thaliana(At, green) andA. arenosa(Aa, red) chromosomes using At and Aa centromeric repetitive sequences as probes, respectively. Five pairs of At chromosomes and eight pairs of Aa chromosomes were present in an F1 allotetraploid, a selfed F8 allotetraploid and naturalA. suecica. Scale bar, 5 μm. (b) Flow chart showing quantification ofcisandtranseffects and classification of the transcripts withcisandtranseffects. (c) Clustered heat map showing transcripts with statistically significant effects of onlycis, onlytrans, and bothcisandtrans. (d) More transcripts withcisthan withtranseffects. The relative expression levels between At and Aa (xaxis) was plotted against the relative expression levels of At and Aa alleles in the F1 allotetraploid. The transcripts with onlycis(green) and onlytrans(red) effects are shown. (e) The relationship between the cumulative number of transcripts (yaxis) and the upper limit of the difference between absolute values ofcisandtranseffects (xaxis). Red and green curves represent the number of transcripts with highertransand higherciseffects, respectively. Figure 1: Arabidopsis allotetraploids progenitors and distribution of genes with cis and trans effects. ( a ) Fluorescence in situ hybridization images of A. thaliana (At, green) and A. arenosa (Aa, red) chromosomes using At and Aa centromeric repetitive sequences as probes, respectively. Five pairs of At chromosomes and eight pairs of Aa chromosomes were present in an F1 allotetraploid, a selfed F8 allotetraploid and natural A. suecica . Scale bar, 5 μm. ( b ) Flow chart showing quantification of cis and trans effects and classification of the transcripts with cis and trans effects. ( c ) Clustered heat map showing transcripts with statistically significant effects of only cis , only trans , and both cis and trans . ( d ) More transcripts with cis than with trans effects. The relative expression levels between At and Aa ( x axis) was plotted against the relative expression levels of At and Aa alleles in the F1 allotetraploid. The transcripts with only cis (green) and only trans (red) effects are shown. ( e ) The relationship between the cumulative number of transcripts ( y axis) and the upper limit of the difference between absolute values of cis and trans effects ( x axis). Red and green curves represent the number of transcripts with higher trans and higher cis effects, respectively. Full size image A. thaliana reads were mapped against A. thaliana genome and complementary DNA sequence databases (TAIR9). A single-nucleotide polymorphism (SNP) database was developed between A. thaliana (At) and A. arenosa (Aa) genes, using two RNA-seq libraries from leaves and siliques, a normalized library from all tissues including flowers, and a large pool of genomic reads, all from A. arenosa . The SNP table included 1,302,037 SNPs with an average of 58 SNPs per gene ( Supplementary Data 1-5 ), which was used to map A. arenosa reads and discriminate between homoeologous transcripts in allotetraploids into At and Aa homoeologous loci or alleles. For simplicity, in this study, the term homoeologous loci and alleles are used interchangeably, so are the F1 interspecific hybrid and F1 allotetraploid. To ensure the accuracy of discrimination between At and Aa homoeologous alleles in allotetraploids, only transcripts with 20 or more SNPs between At and Aa were included in the read assignment. In a simulation test, using the SNPs to assign the reads that were randomly selected from the parental (At or Aa) pools, the proportion of the correctly assigned At reads was relatively higher than Aa reads ( Supplementary Fig. S2a ). This is because DNA polymorphism levels are higher in A. arenosa than in A. thaliana populations [23] . As a result, more A. thaliana than A. arenosa reads are mappable using the SNP database (Methods). To correct this bias, we established a relationship between the expected and predicted allelic values for each gene, by using the simulated dataset with expected allelic values and linear regression analysis ( Supplementary Fig. S2b ). After correction, the allelic expression level was calculated as reads per kilobase of exon model per million (RPKM) using all mapped reads [24] . Variation of cis - and trans -regulation can be distinguished by allelic expression ratios between the parents relative to an F1 interspecific hybrid or allotetraploid ( Fig. 1b ). The expression divergence between species is caused by a combination of both cis and trans effects ( A =log 2 (At/Aa)). In the F1 hybrid, because two alleles were in the same cell, trans expression difference between two parental genes would be eliminated. Therefore, the relative expression differences between At and Aa homoeologs in the F1 hybrid would reflect cis effects ( B =log 2 (F1At/F1Aa)) [12] , [13] . Consequently, trans effects ( A – B ) could be estimated by subtracting cis effects ( B ) from cis and trans effects ( A ). Specifically, the alleles that were expressed differently between the parents and remained differentially expressed in the F1 hybrid ( A = B ) were classified as only cis effects ( Fig. 1b,c,d , green; Supplementary Fig. S3a ), whereas the alleles that were expressed differently between the parents, but equally in the interspecific hybrid ( B =0 and A ≠ B ), were classified as only trans effects ( Fig. 1b,c,d , red; Supplementary Fig. S3b ). Otherwise, cis and trans effects ( cis – trans ) were co-acting. Notably, additional variables in the formula may affect estimating trans effects, and underestimation of the variance could be larger in the trans effect than in the cis effect, which may lead to a potential overestimation of trans effects. After excluding the genes with low expression levels (for example, transcripts with RPKM ≤2) or genes with high sequence identity between At and Aa (that is, low SNP coverage), we identified 14,713 transcript units (corresponding to 11,018 genes with 3,695 alternatively spliced transcripts) that showed allelic expression with statistical significance in the F1 (Methods). Among these transcripts, 2,775 (~18.9%) and 1,139 (~7.7%) were associated with only cis and only trans effects, respectively, and 747 (~5.1%) transcripts were associated with both cis and trans effects ( cis – trans ) ( Fig. 1c,d and Supplementary Data 6 ). The remaining 10,052 (~68.3%) transcripts showed no allelic expression difference between the parents or in the F1. The sum of allelic expression divergence (~32%) is consistent with ~40% of differentially expressed transcripts in a microarray study using the per-gene variance analysis without knowing allelic information [7] . The number of transcripts with larger cis effects is ~119% more than that with larger trans effects (Wilcoxon rank-sum test, | cis | > | trans |, P <2.2e-16) ( Fig. 1e ). These data suggest that cis -regulatory changes have a major role in differential gene expression between Arabidopsis species, which is consistent with the data in yeast [12] . Moreover, percentages of the genes with TATA elements were positively correlated with levels of expression divergence, although the genes with TATA boxes were more enriched in trans effects ( R =0.87, P =4.44e-16) than in cis effects ( R =0.72, P =3.70e-09) ( Supplementary Fig. S4 ). This suggests a role for TATA elements in increased levels of cis - and trans -regulation, as observed in yeast hybrids [25] . Interactive cis and trans effects on expression divergence To further understand cis and trans effects on gene-expression divergence between A. thaliana and A. arenosa , we compared the level of expression divergence of 2,775 only cis and 1,139 only trans transcripts with the transcripts without cis or trans effects ( Fig. 2a ). On the basis of per-transcript unit, both only cis and only trans transcripts showed increased levels of expression divergence relative to those without cis or trans effects ( P <2.2e-16). But the transcripts with only cis and only trans effects have similar levels of expression divergence ( P =0.411). Thus, each transcript with only cis or trans effect contributes equally to gene-expression divergence, although there are more transcripts with only cis effects than with only trans effects. 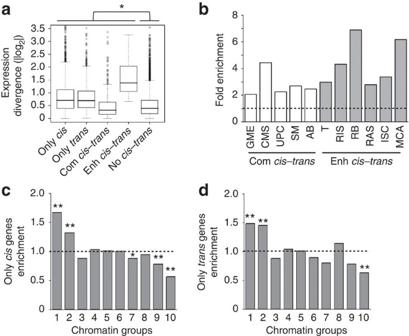Figure 2: Interactions betweencisandtranseffects and enrichment of genes withcisandtranseffects. (a) Relative expression divergence between At and Aa transcripts resulting from onlycis, onlytrans, compensating (Com) and enhancing (Enh)cisandtransinteractions. The control was the expression divergence of transcripts withoutcis–transinteractions. An asterisk indicates a significant difference. (b) Gene ontology enrichment of genes with compensating (white boxes) and enhancing (grey boxes)cisandtransinteractions (P<0.01), relative to the genes in the whole genome (dashed line). GME, Generation of metabolite precursors and energy; CMS, cellular metabolites salvage; UPC, ubiquitin-dependent protein catabolism; SM, sulfur metabolism; AB, amine biosynthesis; T, translation; RIS, response to inorganic substance; RB, ribosome biogenesis; RAS, response to abiotic stimulus; ISC, intracellular signaling cascade; MCA, macromolecular complex assembly. (c) Enrichment of onlycisgenes compared with all genes (dashed line) in ten chromatin groups26(xaxis). (d) Enrichment of onlytransgenes compared with all genes (dashed line) in ten chromatin groups26(X-axis). Asterisks (* and **) indicate the significant levels of 0.05 and 0.01, respectively (χ2test). Figure 2: Interactions between cis and trans effects and enrichment of genes with cis and trans effects. ( a ) Relative expression divergence between At and Aa transcripts resulting from only cis , only trans , compensating (Com) and enhancing (Enh) cis and trans interactions. The control was the expression divergence of transcripts without cis – trans interactions. An asterisk indicates a significant difference. ( b ) Gene ontology enrichment of genes with compensating (white boxes) and enhancing (grey boxes) cis and trans interactions ( P <0.01), relative to the genes in the whole genome (dashed line). GME, Generation of metabolite precursors and energy; CMS, cellular metabolites salvage; UPC, ubiquitin-dependent protein catabolism; SM, sulfur metabolism; AB, amine biosynthesis; T, translation; RIS, response to inorganic substance; RB, ribosome biogenesis; RAS, response to abiotic stimulus; ISC, intracellular signaling cascade; MCA, macromolecular complex assembly. ( c ) Enrichment of only cis genes compared with all genes (dashed line) in ten chromatin groups [26] ( x axis). ( d ) Enrichment of only trans genes compared with all genes (dashed line) in ten chromatin groups [26] (X-axis). Asterisks (* and **) indicate the significant levels of 0.05 and 0.01, respectively (χ 2 test). Full size image Cis and trans effects could act in the same direction (enhancing cis and trans ) or in opposite directions (compensating cis and trans ) in governing their gene expression ( Fig. 1b ). Stabilizing selection would reduce gene-expression divergence between species, resulting in compensating cis and trans effects [12] . On the contrary, disruptive or diversifying selection would promote gene-expression divergence, leading to enhancing cis and trans effects. Among 747 transcripts with significant cis and trans effects ( Fig. 1b,c ), 677 (~91%) were subject to compensating cis – trans interactions, and only 70 (~9%) were related to enhancing cis–trans interactions ( Supplementary Data 6 ). Expression divergence of the transcripts with enhancing cis and trans interactions was significantly higher than that with compensating cis and trans interactions. ( Fig. 2a ) ( P <2.2e-16). Moreover, transcripts with compensating cis and trans interactions showed lower levels of expression divergence than the transcripts without cis and trans effects ( Fig. 2a ) ( P =0.041). These data suggest a prevalent role for stabilizing selection in the genes with compensating cis – trans interactions between species. Gene ontology analysis indicated that genes with enhancing cis and trans interactions were associated with stresses and response to inorganic substances. In contrast, genes with compensating interactions were associated with biosynthetic and metabolic processes ( Fig. 2b ). Conserved expression of genes associated with synthesis of cellular metabolites is likely advantageous for an organism to maintain growth and developmental stability, whereas increased expression divergence of stress- and signaling-responsive genes may enhance the ability of an organism to respond to environmental cues and adapt to ecological niches. Evolutionary fate of the genes with expression divergence could result from selective pressure acting on protein-coding sequences, which can be estimated by nonsynonymous and synonymous substitution ratios ( K a/ K s= ω ). For A. arenosa cDNAs, we assembled short reads and analysed those that contained 75% or more of complete cDNA sequences. For the genes subjected to only cis or only trans effects, more than 99% of genes have K a/ K s values less than one, suggesting purifying selection ( Supplementary Data 7 ). The correlation between K a/ K s values and expression divergence for the genes with only cis effects is statistically significant ( R 2 =0.011, P =3.511e-06), although this correlation for the genes with only trans effects was not significant ( R 2 =0.004, P =0.086) ( Supplementary Table S2 ). The data suggest that coding sequences of the genes with only cis effects and lower levels of expression divergence are subjected to more stringent negative selection than those with higher levels of expression divergence. In addition, K a/ K s values of the genes with enhancing and compensating cis and trans effects were less than one. The difference of K a/ K s values between genes with compensating and enhancing interactions was not statistically significant ( P =0.489), suggesting that purifying selection has relatively equal impact on the genes with enhancing and compensating cis and trans effects. Role of chromatin modifications in cis and trans effects Chromatin regulators and epigenetic effects are predicted to have a role in trans effects as well as cis and trans interactions [11] . In A. thaliana , distinct chromatin modification groups for genes with different histone modifications were defined, using chromatin immunoprecipitation coupled with sequencing (ChIP-seq) and microarrays (ChIP-chip) [26] , [27] . Compared with all transcripts, transcripts with only cis or only trans effects were significantly enriched in chromatin groups 1 and 2 (G1 and G2) ( Fig. 2c,d ). Both G1 and G2 genes are associated with high levels of H3K9 acetylation and H3K4 trimethylation but differ in the variance of expression and histone mark distribution levels [26] . The genes with cis and trans effects were significantly underrepresented in G10 that had high levels of H3K27 trimethylation and low levels of expression. The genes with cis but not trans effects were underrepresented in G9 that was associated with DNA methylation, which predominantly occurs at heterochromatin and repetitive elements such as transposons. The genome-wide chromatin data are consistent with the experimental data in which protein-coding genes and transposons are epigenetically modified in allopolyploids of Arabidopsis [28] , [29] , [30] , [31] and wheat [32] . These data collectively support a role for chromatin modifications in cis and trans regulation of allelic expression divergence between A. thaliana and A. arenosa . Dominance of A. arenosa trans factors in allelic expression Trans -acting factors could bind cis -regulatory regions of homoeologous alleles in a trans- acting manner and such binding could have different effects on expression between two homoeologous alleles in an interspecific hybrid or allotetraploid ( Supplementary Fig. S5 ). An A. thaliana trans factor would lead to equal expression of the same ( cis -acting) At allele between A. thaliana and F1, whereas an A. arenosa trans factor would result in equal expression of the same ( cis -acting) Aa allele between A. arenosa and F1 ( Supplementary Data 8 ). We selected 1,886 transcripts that are subjected to either only trans or cis – trans effects and investigate the roles for At and Aa trans factors in causing allelic expression difference in F1 allotetraploids and their parents. In the F1 allotetraploids, more Aa alleles than At alleles displayed low levels of expression divergence between F1 allotetraploids and their parents ( Fig. 3a ). In contrast, more At alleles than Aa alleles showed high levels of expression difference between F1 allotetraploids and their parents (paired t -test, P <2.2e -16). The data suggest that A. arenosa trans -acting factors have greater effects than A. thaliana ones on allelic gene-expression difference between F1 allotetraploids and their parents, consistent with the overall expression dominance of A. arenosa genes over A. thaliana genes [7] . 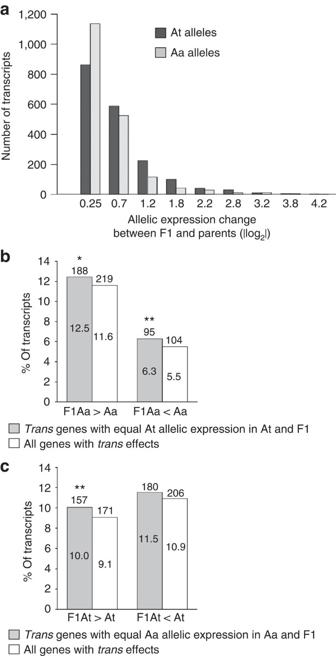Figure 3: Effects of At and Aatrans-acting factors on up- and down-regulation of At and Aa alleles in F1 allotetraploid. (a) A relationship between the number of transcripts withtranseffects (yaxis) and absolute values of allelic expression difference between F1 allotetraploid andA. thalianaorA. arenosa(xaxis). More At than Aa alleles showed a high level of expression difference, whereas more Aa than At alleles displayed a low level of expression difference. (b–c) The relationship between the proportion of transcripts (yaxis) with up- (left) or down- (right) regulated Aa alleles (b) or At alleles (c) between F1 allotetraploid and the respective parent (xaxis). Transcripts with equal At allelic expression between At and F1 (b) and transcripts with equal Aa allelic expression between Aa and F1 (c) were compared with all transcripts withtranseffects, respectively. The expression differences were caused by Attrans-acting factors (b) or Aatrans-acting factors (c). The numbers above and within each bar represents the number and percentage of transcripts, respectively. Asterisks (* and **) indicate significant levels of 0.05 and 0.01, respectively (χ2test). Figure 3: Effects of At and Aa trans -acting factors on up- and down-regulation of At and Aa alleles in F1 allotetraploid. ( a ) A relationship between the number of transcripts with trans effects ( y axis) and absolute values of allelic expression difference between F1 allotetraploid and A. thaliana or A. arenosa ( x axis). More At than Aa alleles showed a high level of expression difference, whereas more Aa than At alleles displayed a low level of expression difference. ( b–c ) The relationship between the proportion of transcripts ( y axis) with up- (left) or down- (right) regulated Aa alleles ( b ) or At alleles ( c ) between F1 allotetraploid and the respective parent ( x axis). Transcripts with equal At allelic expression between At and F1 ( b ) and transcripts with equal Aa allelic expression between Aa and F1 ( c ) were compared with all transcripts with trans effects, respectively. The expression differences were caused by At trans -acting factors ( b ) or Aa trans -acting factors ( c ). The numbers above and within each bar represents the number and percentage of transcripts, respectively. Asterisks (* and **) indicate significant levels of 0.05 and 0.01, respectively (χ 2 test). Full size image For genes with only trans effects, expression difference between a homoeologous allele (for example, Aa allele) in the F1 allotetraploid, and its corresponding parent (for example, A. arenosa ) is likely caused by the presence of the homoeologous trans factors from the other parent (for example, At trans factor) ( Supplementary Fig. S5 ). Compared with all genes with trans effects, a proportion of Aa alleles in the F1 allotetraploid was either upregulated (12.5%, Chi-squared test P =0.027) or down-regulated (6.3%, Chi-squared test P =0.004) by A. thaliana trans -factors ( Fig. 3b ). For At alleles, such enrichment (10%, χ 2 test P =0.002) was only observed for genes that were upregulated by A. arenosa trans -factors ( Fig. 3c ). These data suggest that A. thaliana trans- factors act as both activators and repressors for expression of Aa alleles in F1 allotetraploids. In contrast, A. arenosa trans- factors are more like to cause upregulation of At alleles in F1 allotetraploids. This notion is supported by available experimental data. As examples, the A. thaliana L er genome in allotetraploids contains a non-functional FRIGIDA (FRI), and the A. arenosa FRI trans -activates expression of homoeologous A. thaliana FLOWERING LOCUS C , leading to later flowering [28] . A. arenosa miR163 is more downregulated than A. thaliana miR163 in allotetraploids [33] . For many genes involved in photosynthesis, starch metabolism and circadian pathways, A. thaliana alleles are preferentially upregulated in the allotetraploids, leading to hybrid vigour [29] . Transmission of allelic expression in allotetraploids In Arabidopsis -resynthesized F1 and F8 allotetraploids, cis -regulatory changes are negligible [7] , [28] ; allelic expression variation is mainly caused by epigenetic changes [5] , leading to trans effects as well as cis and trans interactions. To test whether the effects of parental cis and trans regulatory changes in F1 are persistent over generations, we compared allelic expression changes in F1, F8 and the natural A. suecica that was formed between extant A. thaliana and A. arenosa [23] . Among three allotetraploids lines (F1, F8 and As), expression of At or Aa alleles showed the strongest correlation between F1 and F8 allotetraploids ( R 2 =0.86 for At and 0.84 for Aa), followed by those between F8 and As ( R 2 =0.64 for At and 0.61 for Aa) and between F1 and As allotetraploids ( R 2 =0.59 for both At and Aa) ( Fig. 4a , Supplementary Data 9 , Supplementary Table S3 and Supplementary Fig. S6 ). Moreover, the overall expression correlation between homoeologous At and Aa alleles within the F1, F8 or As allotetraploids were relatively high ( R 2 =0.63 to 0.79). The strongest correlation was observed in F1 ( R 2 =0.79), followed by that in F8 ( R 2 =0.71) and As ( R 2 =0.63) allotetraploids. Such trend is consistent with increased expression ratios between At–Aa homoeologs from F1 and F8, to As allotetraploids ( Fig. 4b ). Collectively, these data indicate a rapid establishment of homoeologous gene-expression program in the F1 allotetraploids, immediately after interspecific hybridization [21] . Moreover, increase in the expression difference between At–Aa homoeologs from F1 and F8 to As suggests cis- regulatory changes in At or Aa alleles during allotetraploid evolution. 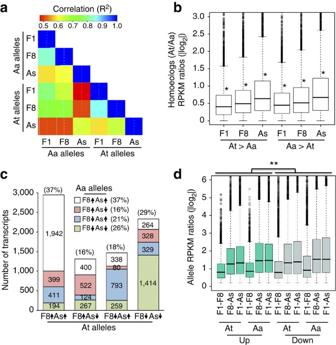Figure 4: Correlation of allelic expression in F1, F8 and naturalA. suecica. (a) Heat map of expression correlations between At and Aa alleles in F1, F8 and naturalA. suecica. Correlation coefficient (R2) is showed in colour scale to reflect the strength of association between two comparisons. (b) Box and whisker plots showing expression divergence between homoeologs (RPKM ratios) in F1, F8 or As allotetraploids with a significant level (P-value < 0.001 and *). (c) The number of transcripts (yaxis) showing At and Aa allelic expression changes in F8 and As relative to F1. Numbers indicate proportions of Aa alleles with expression (relative to F1) that are up in both F8 and As (white), up in F8 and down in As (red), down in F8 and up in As (blue), and down in both F8 and As (green). The same four classifications of At alleles were showed inxaxis. The number and percentage (in parenthesis) of transcripts in each expression combination are showed. (d) Box and whisker plots showing the relationship between absolute values of RPKM ratios (yaxis) and up- or down-regulation of At and Aa alleles in various F1, F8 and naturalA. suecicacomparisons. A cutoff of 0.1 |log2| ratio was used to define transcripts with up- or down-regulation with a significant level (P-value < 2.1e-06 and **). Figure 4: Correlation of allelic expression in F1, F8 and natural A. suecica . ( a ) Heat map of expression correlations between At and Aa alleles in F1, F8 and natural A. suecica . Correlation coefficient ( R 2 ) is showed in colour scale to reflect the strength of association between two comparisons. ( b ) Box and whisker plots showing expression divergence between homoeologs (RPKM ratios) in F1, F8 or As allotetraploids with a significant level ( P -value < 0.001 and *). ( c ) The number of transcripts ( y axis) showing At and Aa allelic expression changes in F8 and As relative to F1. Numbers indicate proportions of Aa alleles with expression (relative to F1) that are up in both F8 and As (white), up in F8 and down in As (red), down in F8 and up in As (blue), and down in both F8 and As (green). The same four classifications of At alleles were showed in x axis. The number and percentage (in parenthesis) of transcripts in each expression combination are showed. ( d ) Box and whisker plots showing the relationship between absolute values of RPKM ratios ( y axis) and up- or down-regulation of At and Aa alleles in various F1, F8 and natural A. suecica comparisons. A cutoff of 0.1 |log2| ratio was used to define transcripts with up- or down-regulation with a significant level ( P -value < 2.1e-06 and **). Full size image We next analysed the directions of allelic expression changes from F1 to F8 and to As allotetraploids ( Fig. 4c ; Supplementary Table S4 ). For alleles with the same directional expression change in F8 and As, 37% of At (2,946/ 8,064) or Aa (2,944/ 8,064) alleles were upregulated whereas 29% of At (2,335/ 8,064) and 26% of Aa (2,134/ 8,064) alleles were downregulated. This indicates that two-thirds (65 and 63% for At and Aa alleles, respectively) of allelic expression changes were in the same direction. Approximately one-third of allelic expression changes (34 and 37% for At and Aa alleles, respectively) were in the opposite direction between F8 and As. Between At and Aa homoeologs, ~58% showed concerted up- or down-regulation in F8 and As relative to F1. For examples, among 2,335 At alleles that were downregulated in both F8 and As, 1,414 Aa alleles were also downregulated. And for 1,470 At alleles with downregulation in F8 and upregulation in As, 793 Aa alleles also showed the same trend of expression changes. In contrast, At and Aa homoeologs with expression changes in the opposite directions accounted for the lowest portion in each comparison. For example, among 2,946 At alleles that were upregulated in both F8 and As, 194 of the Aa alleles were downregulated, accounting for only 7% within that group. Overall, only 8% of homoeologs in all four categories showed expression changes in opposite directions. These concerted expression changes in homoeologous loci, during evolution of allotetraploids, are likely caused by trans -acting factors because simultaneous changes in cis -regulatory elements of genes originating from both progenitor species are less likely. Although the total number of upregulated At or Aa alleles was higher than that of downregulated alleles in F1, F8 and As ( Fig. 4c ), the level of expression divergence for downregulated alleles was consistently higher than that of upregulated alleles ( Fig. 4d , t -test, P <2.1e-06). This may explain the difference in the number of genes detected between RNA-seq and microarray experiments, because microarrays often detect the genes with high expression levels. Moreover, the level of expression divergence of At or Aa alleles, regardless of up- or down-regulated, was the lowest between F1 and F8. For At alleles, expression divergence of up- and down-regulation was the higher between F1 and As than between F8 and As. For Aa alleles, upregulated alleles showed the highest level of expression divergence between F8 and As, whereas downregulated alleles displayed the highest level of expression divergence between F1 and As ( Fig. 4d ). Higher levels of allelic expression divergence between A. suecica and F1 than between As and F8 may result from a high level of heterozygosity in A. arenosa . Our data suggest a model for cis and trans effects on genes expression divergence between Arabidopsis -related species and their allotetraploids ( Fig. 5a,b ). Gene-expression divergence in allopolyploids or interspecific hybrids and their progenitors is predicted to involve epigenetic factors and genetic changes including sequence divergence and mutations [5] . At the epigenetic level, chromatin modifications and other epigenetic factors are predicted to alter cis and trans regulation [11] . In the medaka fish genome, a distinctive pattern of ~200-bp periodic sequence changes, downstream of transcription start sites, is correlated with the chromatin structure [34] . In the human genome, synonymous substitution rate at non-CpG sites is the highest in regions of the open chromatin [35] , linking cis effects with chromatin structure. On the other hand, trans expression variability is largely affected by chromatin factors, which have more important roles in creating regulatory variation than transcription factors [36] . Our experimental data suggest that both cis and trans effects are associated with genes that are enriched with H3K9 acetylation and H3K4 trimethylation [26] . Cis but not trans effects are underrepresented in the genes and elements associated with DNA methylation, suggesting that these DNA elements including transposons are likely controlled by trans factors. These factors could include chromatin remodellers and small RNAs, which induce RNA-directed DNA methylation [37] . This could be tested using sequencing analysis of small RNAs and methyl-cytosine in these species. 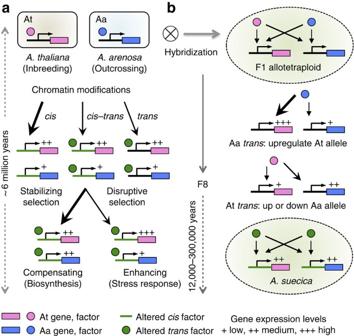Figure 5: Model forcisandtranseffects on genes expression changes inArabidopsisallotetraploids and their progenitors. (a) Possible modes ofcis,transandcisandtrans(cis–trans) interactions leading to gene-expression divergence betweenA. thaliana(At) andA. arenosa(Aa) that diverged ~6 million years ago22. Fat arrows indicate predominantciseffects overtransorcis–transeffects and stabilizing selection over disruptive selection forcis–transeffects. As a result, either At (shown in the diagram) or Aa alleles could increase expression levels. (b) Possible modes of At and Aa allele interactions leading to homoeologous genes expression changes within F1 allotetraploids, among allotetraploid lineages (F8), and a natural allotetraploid (A. suecica) that was formed 12,000–300,000 years ago41. Aatransfactors tended to upregulate At alleles, whereas Attransfactors tended to either up- or down-regulate Aa alleles. The majority of At and Aa alleles tended to change their expression into the same direction. As a result, At and Aa allele could have the same or different levels of expression (Aa > At, shown in the diagram). Box and circle represent genes andtransregulators, respectively. Red and blue indicate At and Aa genes and factors, respectively. Black line attached to the box (gene) indicateciselements in At or Aa. Green lines and circles indicate alteredciselements andtransfactors, respectively. Figure 5: Model for cis and trans effects on genes expression changes in Arabidopsis allotetraploids and their progenitors. ( a ) Possible modes of cis , trans and cis and trans ( cis – trans ) interactions leading to gene-expression divergence between A. thaliana (At) and A. arenosa (Aa) that diverged ~6 million years ago [22] . Fat arrows indicate predominant cis effects over trans or cis – trans effects and stabilizing selection over disruptive selection for cis – trans effects. As a result, either At (shown in the diagram) or Aa alleles could increase expression levels. ( b ) Possible modes of At and Aa allele interactions leading to homoeologous genes expression changes within F1 allotetraploids, among allotetraploid lineages (F8), and a natural allotetraploid ( A. suecica ) that was formed 12,000–300,000 years ago [41] . Aa trans factors tended to upregulate At alleles, whereas At trans factors tended to either up- or down-regulate Aa alleles. The majority of At and Aa alleles tended to change their expression into the same direction. As a result, At and Aa allele could have the same or different levels of expression (Aa > At, shown in the diagram). Box and circle represent genes and trans regulators, respectively. Red and blue indicate At and Aa genes and factors, respectively. Black line attached to the box (gene) indicate cis elements in At or Aa. Green lines and circles indicate altered cis elements and trans factors, respectively. Full size image Although both cis and trans effects contribute to expression divergence between species, there are more genes with cis effects than those with trans effects. However, on a per-gene basis, cis and trans effects on the level of expression divergence are similar. For genes subjected to both cis and trans effects, expression divergence maintained by cis effects could be eliminated by compensating trans effects, resulting in convergence of gene expression originating in the parents (stabilizing selection). As examples, ribosomal proteins are significantly enriched in the compensating cis and trans genes ( P =2.7e-05). In yeast, cis elements of ribosomal protein genes are highly divergent between Saccharomyces cerevisiae and Candida albicans [38] . Moreover, transcription factors affect expression evolution of ribosomal proteins [39] . These data suggest a role for cis and trans interactions in the ribosome regulation. At the gene function level, compensating cis and trans interactions drive expression divergence of genes involving metabolic and biosynthetic processes into similar expression levels, leading to the stability of internal cellular functions. Plants have to respond the ever-changing environment, and the genes associated with abiotic stimuli are influenced by enhancing cis and trans effects that are under disruptive selection, which increases levels of gene-expression diversity. In F1 allotetraploids, A. arenosa trans regulators have larger (or dominant) effects than A. thaliana trans factors on allelic expression divergence, and trans regulators tend to reduce expression divergence between homoeologous alleles ( Fig. 5b ). A high level of sequence variation within A. arenosa population [23] may confer plasticity of trans factors for their binding to interacting factors and cis elements originating from a related species. In contrast, natural A. thaliana is an inbred diploid [20] . A high level of homozygosity, caused by inbreeding, is predicted to increase the specificity of interactions between trans factors and cis -elements. In allotetraploids, an A. arenosa trans factor is predicted to bind heterologous cis elements. Moreover, interactions between Aa trans factors and cis elements of At alleles or vice versa result in up- or down-regulation of At and Aa alleles. This may explain at least in part why different dominant expression patterns were identified in the same [8] , [40] or different allopolyploids [7] . Although two-thirds of allelic expression changes are in the same direction between resynthesized A. suecica -like allotetraploids and natural A. suecica lines, one-third of alleles show expression changes in different directions. Moreover, the majority (~58%) of At and Aa allelic expression changes are in the same direction from F1 to F8 and natural A. suecica lines, supporting a notion of dominant trans regulatory changes during selfing. A. suecica had a single origin at 12,000–300,000 years ago [41] . Combination of predominant cis effects between species and predominant trans effects during selfing might act in concert to provide opportunities for new allopolyploids to increase levels of adaptation and diversification during evolution [3] , [4] . A higher level of gene-expression divergence between F1 allotetraploids and A. suecica may suggest that many genes have diverged their expression over time. These data collectively provide evidence for roles of epigenetic and genetic regulation in allelic expression divergence and transgenerational inheritance of cis and trans regulation and growth vigor that are associated with hybrids and allopolyploids, including many important agricultural crops. Plant materials and growth conditions Plant materials include A. thaliana autotetraploids (At; ABRC, CS3900), A. arenosa (Aa; ABRC, CS3901), F1 resynthesized allotetraploids (AlloF1), F8 allotetraploids (AlloF8; ABRC, CS3895), and a natural allotetraploid A. suecica . All plants were grown under a 16/8-h light/dark cycle with temperatures of 22 °C (light) and 20 °C (dark). Rosette leaves before bolting (flowering) were collected for DNA and RNA analysis. Fluorescence in situ hybridization Fluorescence in situ hybridization was performed according to the published protocols with modifications [42] , [43] . In brief, floral buds (At4, Aa, AlloF1 and AlloF8) were fixed in ice-cold Carnoy's fixative for at least 1.5 h. Selected floral buds (<1 mm) were digested in a pectolytic enzyme mixture (0.3% cellulase, 0.3% pectolyase and 0.3% cytohelicase) for 2 h. After digestion, cells were suspended in 9:1 glacial acetic acid:methanol, and one drop of cell suspension was placed on a glass slide. Chromosomal DNA was crosslinked to slides by exposure to ultraviolet light in Stratalinker UV Crosslinker 2400 (120 mJ cm −2 ) (Stratagene, Santa Clara, CA, USA). Centromeric repetitive sequences of At4 (AtCEN) and Aa (AaCEN) were amplified by PCR, using genomic DNA as template and the primers as previously described [44] . PCR products were purified using QIAquick PCR Purification Kit (Qiagen, Valencia, CA, USA). One microgram of purified AtCEN and AaCEN PCR products were labelled with Fluorescein-12-dUTP (Fermentas, Glen Burnie, MD, USA) and Texas red-5-dCTP (Perkin Elmer, Waltham, MA, USA), respectively, using the nick-translation method. Labelled probes were purified using MinElute PCR Purification Kit (Qiagen). Hybridization of chromosome mounts was performed at 55 °C for 4–6 h in the presence of the labelled probes. Vectashield Mounting Medium with DAPI (Vector Laboratories, Burlingame, CA, USA) was applied to hybridized slides before observation. Images were taken using a Zeiss Axiovert 200 M microscope equipped with a Zeiss Axiocam fluorescence camera, and processed using Adobe Photoshop 7.0. mRNA-seq library preparation Total RNA was isolated from mature leaves (3–4 week-old A. thaliana ; 6–7-week old A. arenosa or allotetraploids plants) before bolting using plant RNA purification reagent (Invitrogen, Carlsbad, CA, USA). The integrity of extracted RNA was verified by resolving 1 μg RNA in a 1% formaldehyde denaturing agarose gel. An aliquot of 10 μg total RNA was used to prepare mRNA-seq libraries using Illumina mRNA-seq sample preparation kit (Illumina, San Diego, CA, USA). Libraries with a range of 200±25 bp were excised and amplified for subsequent cluster generation and massively parallel sequencing using the Illumina Genome Analyzer GII or HiSeq 2000 with read lengths ranged from 38 to 100 bp. Read mapping and expression quantification mRNA-seq reads from 11 libraries ( Supplementary Table S1 ), including three replicates for each of At, Aa and F1, and one replicate for F8 or As, were mapped to TAIR9 genome and cDNA sequence using BFAST software ( http://bfast.sourceforge.net ) [45] . Both unique and multiple best-mapped reads were collected to estimate the expression. Transcript levels were quantified by counting RPKM [24] . We followed procedure of Mortazavi et al . [24] to compute RPKM. First, all unique reads without alternative splice isoforms were used to calculate a preliminary RPKM. Second, unique reads with isoform exons were weighted using the preliminary RPKM. Final RPKMs were calculated by combining the unique and weighted-multiple mapped reads. The RNA-sequence data has been deposited at GEO http://www.ncbi.nlm.nih.gov/geo/ with the accession number GSE29687 . SNPs between A . thaliana and A . arenosa Mappable reads from A. thaliana (At) and A. arenosa (Aa) were aligned onto the A. thaliana reference genome (TAIR9) to identify At and Aa orthologues. These alignments were used to detect SNPs between two ortholgous loci. We restricted the qualified SNPs to those that contained at least two reads in each species. An additional mRNA-seq data set from Aa siliques was included to improve SNPs detection between At and Aa genes. In addition, another SNP dataset derived from diploid At (Col) RNA and normalized Aa mRNAs was kindly provided by Luca Comai at the University of California, Davis. For this SNP dataset, Aa contig sequences were used when constructing the dataset. A comprehensive SNP dataset ( Supplementary Data 1–5 ) integrating all these available resources was used for estimating allelic frequencies in allotetraploids and their progenitors. Allelic expression frequencies in allotetraploids We assigned the reads in an allotetraploids into At and Aa reads, using two or more distinct SNPs between A. thaliana (At) and A. arenosa (Aa). Reads with ambiguous SNP information were excluded. The frequency of allelic expression in an allotetraploid was estimated by the proportion of uniquely mapped At and Aa reads in each locus. Using this method, we tested allele distribution patterns in two parents (At and Aa) by calculating the proportion of randomly selected reads assigned to each genotype. If there is no bias, all reads from At library should be assigned to At alleles, and all reads from Aa library should be assigned to Aa alleles. Results of a simulation test showed that 98.5% of At genes tested each had 90% or more reads with correct read assignment, whereas 72.2% of Aa genes tested each had 90% or more reads with correct read assignment ( Supplementary Fig. S2a ). The percentage of read assignment based on the SNP table was higher for the At than for the Aa reads. To correct this systematic bias, we used a simulation model to generate a relationship between the known allele frequency (expected value) and predicted frequency estimation (predicted value). We selected At and Aa genes each containing at least 20 SNPs and tested three expected expression ratios (At/Aa). The uniquely mapped At and Aa reads were mixed in the ratios of 3:1, 1:1, and 1:3. After nine simulation analyses (3 types of frequencies ×3 simulations per frequency type), nine sets of expected vs predicted frequencies were obtained for each gene. Both linear and quadratic regression analyses were used to calculate the relationship between the two numerical variables, expected and predicted allele frequencies. The data fitted better with the linear regression than with the quadratic curve. Thus, the predicted allelic expression frequency (unique reads per gene) of a gene in allotetraploids was imported into a linear function of the simulation to calculate the expected value. The allelic expression frequency was then converted into an RPKM value [24] , by multiplying with overall RPKM value of each locus. Genes with the RPKM below two were excluded from analysis. Genes of cis and trans effects in A. thaliana and A. arenosa Log 2 -transformed ratios were used to estimate allelic expression divergence. Gene-expression divergence ( A ) between species was computed by log 2 (At/Aa). Cis effects ( B ) were estimated by log 2 (F1At/F1Aa), and trans effects were derived by subtracting cis effects from the expression divergence between species ( A – B ) [12] . Student's t -tests were used to test for differences between At and Aa allelic expression in F1 ( cis effects), as well as differences between parental expression ratio and allelic expression ratio ( trans effects). We employed SGoF program to perform multiple testing correction [46] ( γ =0.05). If a gene showed different expression between parents (At and Aa) but same allelic expression within the hybrid, expression divergence of the gene in parents was considered to be caused by only trans effects. A gene was considered having only cis effects, if the ratio of interspecies allelic expression was equal to the allelic expression in hybrid or allotetraploid ( A = B ). Compensating and enhancing cis and trans interactions We identified compensating and enhancing cis and trans interactions by comparing the directions of cis and trans effects. A compensating cis – trans interaction was implied if cis and trans effects of one gene were in the opposite directions [{ B > 0 and ( A − B ) > 0} or { B <0 and ( A − B ) > 0}]. In contrast, if cis and trans effects of one gene acted in the same direction [{ B > 0 and ( A − B ) > 0} or { B <0 and ( A − B ) < 0}], the interaction was enhancing cis – trans . Accession codes: The RNA-sequence data have been deposited in the Gene Expression Omnibus database under the accession code GSE29687 . How to cite this article: Shi, X. et al . Cis - and trans -regulatory divergence between progenitor species determines gene-expression novelty in Arabidopsis allopolyploids. Nat. Commun. 3:950 doi: 10.1038/ncomms1954 (2012).